Interferon regulatory factor 1 (IRF-1) promotes intestinal group 3 innate lymphoid responses duringCitrobacter rodentiuminfection 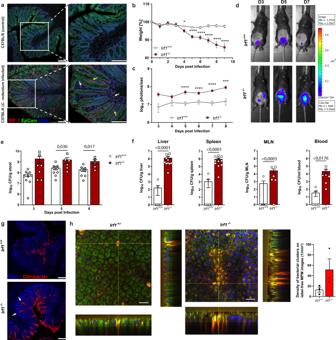Fig. 1: IRF-1 expression is essential to mount efficient C. rodentium directed immunity. aColonic cross sections of uninfected orC. rodentium(9 dpi) infected C57BL/6 mice stained with anti-IRF-1 (red), anti-Ep-CAM (green), and DAPI (blue) and analyzed by confocal microscopy (epithelium: yellow arrow heads; lamina propria cells: white arrow heads). Scale bars represent 100 µm.b–gIrf1+/+andIrf1–/–mice were infected orally with 4 × 109CFU ofC. rodentium.bWeights of infected mice were recorded daily and plotted as percentage of baseline (Irf1+/+:n= 19,Irf1–/–n= 18). Day 4 pvalue: 0,0172; pvalues day5-day9: <0.0001.c,dBacterial loads were measured via in vivo imaging (n= 15/group). Day 8pvalue: 0.0008;pvalues day5–day7: <0.0001.eFecal bacterial loads (CFU/g stool) on 3, 5 and 8 dpi. (Irf1+/+:n= 9,Irf1–/–n= 7).fDissemination ofC. rodentiumto livers (Irf1+/+:n= 13,Irf1–/–n= 11), spleens (Irf1+/+:n= 13,Irf1–/–n= 11), mLN (Irf1+/+:n= 8,Irf1–/–n= 6) and blood (Irf1+/+:n= 8,Irf1–/–n= 6) (9 dpi).gC. rodentiumcolonization of the colonic epithelial surface and penetration of the crypt bottom (white arrow heads) was visualized by staining cross sections by immunohistochemistry. Scale bar: 100 µm.hIrf1+/+andIrf1–/–mice (n= 3/group) were infected with aC. rodentiumreporter-strain expressing M-Ruby-II. Tissue samples from distal colon (7 dpi) were analysed by label-free multiphoton microscopy (MPM; excitation at 810 nm) to define densities of bacterial clusters per MPM image (1/mm2). Scale bar: 50 µm. Data is expressed as mean ± SEM. Two-tailed Mann–Whitney U test was used for statistical comparison. In (e) and (f) exactpvalues are provided in the plots. *p≤ 0.05; ***p≤ 0.001; ****p≤ 0.0001. Source data are provided as a Source data file. Group 3 innate lymphoid cells (ILC3s) are crucial mediators of immunity and epithelial barrier function during immune responses against extracellular bacteria. Here, we identify Interferon regulatory factor 1 (IRF-1), a transcription factor previously associated with type 1 immunity, as an essential regulator of intestinal ILC3 accumulation and effector cytokine production. We demonstrate that IRF-1 is upregulated in the context of infection with the enteropathogen Citrobacter rodentium and that its presence is central for anatomical containment and prevention of pathogen dissemination. We furthermore show that IRF-1 is required in order for intestinal ILC3s to produce large amounts of the protective effector cytokine IL-22 early in the course of infection. On a molecular level, our data indicate that IRF-1 controls ILC3 numbers and their activation by direct transcriptional regulation of the IL-12Rβ1 chain, thereby allowing ILCs to physiologically respond to IL-23 stimulation. Complex and tightly regulated immunological networks of both innate and adaptive immune cells provide intestinal homeostasis and, at the same time, confer effective protection against potentially invasive pathogenic threats. Type 3 innate lymphoid cells (ILC3s) are innate immune cells particularly enriched in gut associated lymphoid tissues (GALT) that are increasingly appreciated as gatekeepers of intestinal barrier integrity and immune homeostasis [1] , [2] . ILC3-derived cytokines directly interact with intestinal epithelial cells (IEC) and modulate other immune cell functions to orchestrate tissue reorganization. While they produce cytokines crucial for barrier protection, dysregulated activation of ILC3s can disrupt gut homeostasis and contribute to severe chronic pathologies such as inflammatory bowel disease (IBD) and colorectal cancer [3] . Although ILC3s are generally defined by the expression of the transcription factor RAR-related orphan nuclear receptor gamma t (RORγt), they are a rather heterogeneous group consisting of different subtypes which, in mice, can be broadly distinguished based on their expression of the C-C chemokine receptor type 6 (CCR6) and the natural cytotoxicity receptor (NCR) NKp46 [4] . LTi-like ILC3s express CCR6 and are capable of secreting substantial amounts of IL-22 and IL-17. CCR6 - NKp46 - ILC3s mainly produce IL-22 and were shown to differentiate in inflammatory settings through the Notch-dependent upregulation of Tbet into CCR6 - NKp46 + ILC3s that mainly produce IFN-γ [5] . As a result of IL-12 and IL-18 stimulation, CCR6 - NKp46 + ILC3s downregulate RORγt and develop into Tbet + ex-RORγt ILC3s or ILC1-like cells [6] . It is believed that this phenotypical plasticity allows ILC3s to adaptively switch between inflammatory and homeostatic phenotypes in accordance with the current environmental conditions [7] , [8] . The non-invasive attaching-effacing bacterial pathogen Citrobacter rodentium has been well appreciated as a model to study the processes that lead to the activation of innate and adaptive components of the intestinal immune system [9] and serves as a model of human infections with enteropathogenic E. coli and enterohaemorrhagic E. coli (EPEC/EHEC) and IBD. During the early phase of infection, the cytokine IL-22 is essential to confer host protection and RORγt-expressing group 3 innate lymphoid cells (ILC3) have been identified as a critical cellular source of this cytokine [10] . The transcription factor interferon regulatory factor 1 (IRF-1) is ubiquitously expressed at low basal levels, where it maintains constitutive expression of its target genes. During various infectious diseases, IRF-1 expression in cells is strongly induced by several factors including interferons or pathogen sensors such as TLRs, NLRs and RLRs [11] , [12] . In the human gut, IRF-1 upregulation has been associated with chronic intestinal inflammation [13] , [14] , while studies of Irf1 –/– mice in a mouse model of chemically induced colitis suggested protective roles during intestinal inflammation [15] . However, even though IRF-1 is well-known as an important contributor to immune defense mechanisms at multiple levels, the role of IRF-1 in innate immune responses at mucosal surfaces remains incompletely understood. In this study, we characterize the function of IRF-1 during the early phase of intestinal inflammatory conditions. We demonstrate that IRF-1 is upregulated in the context of enteric infection with the gram negative model organism C. rodentium and is a central regulator of protective mucosal immunity in this model. We show that impaired IL-22 production by ILC3s in Irf1 –/– mice leads to insufficient intestinal immune protection and a lack of anti-bacterial defense during C. rodentium infection. On a molecular level, ILC intrinsic IRF-1 expression is essential for appropriate intestinal ILC3 activation by controlling their capacity to physiologically respond to IL-12 and IL-23 stimulation. IRF-1 expression is essential to mount efficient immune responses against C. rodentium Previous studies in human IBD and models of intestinal inflammation suggested important gut specific roles of IRF-1. Because immunohistochemical stainings demonstrated a profound increase in colonic IRF-1 protein during C. rodentium infection (Fig. 1a , Supplementary Fig. 1A ), we took advantage of this widely utilized model to establish cell type specific functions of IRF-1 during infections with extracellular, noninvasive enteric pathogens. We therefore infected Irf1 -deficient ( Irf1 –/– ) mice with a luminescent C. rodentium strain and compared both the disease outcome and pathogen burden of these mice with Irf1 +/+ controls. While control mice did not lose weight during the course of infection, Irf1 –/– mice substantially lost weight, starting from day four post infection (Fig. 1b ). Notably, starting at 9 to 10 days post infection (dpi), severe disease in Irf1 –/– mice was evident by rapid weight loss and high mortality rates. To monitor bacterial loads during the course of disease in vivo, the pathogen-derived luminescence was measured daily using IVIS-based in vivo-imaging. Interestingly, detected luminescence intensities were significantly higher in Irf1 –/– mice at every time point of analysis (Fig. 1c, d ) and correlated with increased fecal C. rodentium loads analyzed by plating of serially-diluted stool material on selective agar-plates (Fig. 1e ). On day nine post infection, analysis of tissue homogenates from distal organs (liver, spleen and mesenteric lymph nodes (mLNs)) indicated only low systemic pathogen spread in controls, while Irf1 –/– mice displayed high systemic C. rodentium dissemination (Fig. 1f ). C. rodentium typically attaches to superficial enterocytes that line the intestinal lumen, but does not cover IECs at the crypt base [16] . However, specific immunofluorescent staining demonstrated C. rodentium localization deep in colonic crypts of Irf1 –/– mice, whereas, control mice displayed pathogen signals only at the surface of the crypts as expected (Fig. 1g ). To further characterize C. rodentium -induced mucosal lesions, we also used multiphoton microscopy with fresh colonic tissue [17] to visualize infection-induced bacterial foci in infected mice. These experiments further confirmed an increased manifestation of mucosal C. rodentium clusters in Irf1 –/– mice and provided evidence that the absence of IRF-1 allows deep crypt penetration of the pathogen (Fig. 1h ). Fig. 1: IRF-1 expression is essential to mount efficient C. rodentium directed immunity. a Colonic cross sections of uninfected or C. rodentium (9 dpi) infected C57BL/6 mice stained with anti-IRF-1 (red), anti-Ep-CAM (green), and DAPI (blue) and analyzed by confocal microscopy (epithelium: yellow arrow heads; lamina propria cells: white arrow heads). Scale bars represent 100 µm. b – g Irf1 +/+ and Irf1 –/– mice were infected orally with 4 × 10 9 CFU of C. rodentium . b Weights of infected mice were recorded daily and plotted as percentage of baseline ( Irf1 +/+ : n = 19, Irf1 –/– n = 18). Day 4 pvalue: 0,0172; pvalues day5-day9: <0.0001. c , d Bacterial loads were measured via in vivo imaging ( n = 15/group). Day 8 p value: 0.0008; p values day5–day7: <0.0001. e Fecal bacterial loads (CFU/g stool) on 3, 5 and 8 dpi. ( Irf1 +/+ : n = 9, Irf1 –/– n = 7). f Dissemination of C. rodentium to livers ( Irf1 +/+ : n = 13, Irf1 –/– n = 11), spleens ( Irf1 +/+ : n = 13, Irf1 –/– n = 11), mLN ( Irf1 +/+ : n = 8, Irf1 –/– n = 6) and blood ( Irf1 +/+ : n = 8, Irf1 –/– n = 6) (9 dpi). g C. rodentium colonization of the colonic epithelial surface and penetration of the crypt bottom (white arrow heads) was visualized by staining cross sections by immunohistochemistry. Scale bar: 100 µm. h Irf1 +/+ and Irf1 –/– mice ( n = 3/group) were infected with a C. rodentium reporter-strain expressing M-Ruby-II. Tissue samples from distal colon (7 dpi) were analysed by label-free multiphoton microscopy (MPM; excitation at 810 nm) to define densities of bacterial clusters per MPM image (1/mm 2 ). Scale bar: 50 µm. Data is expressed as mean ± SEM. Two-tailed Mann–Whitney U test was used for statistical comparison. In ( e ) and ( f ) exact p values are provided in the plots. * p ≤ 0.05; *** p ≤ 0.001; **** p ≤ 0.0001. Source data are provided as a Source data file. Full size image We next used RNAseq-based gene expression profiling to investigate the impact of IRF-1 inactivation on the global colonic transcriptome in whole colonic tissue of mice with C. rodentium infection. Thereby, unsupervised hierarchical clustering of normalized gene expression counts showed high similarities in transcriptional patterns within each experimental group, but substantial differences between the two experimental groups. (Fig. 2a ). Accordingly, more than 1000 genes were differentially expressed between Irf1 –/– and Irf1 +/+ mice (log2 fold change >2; p < 0.05). While the majority of these genes was downregulated in Irf1 –/– mice (681 out of 1023), 342 were upregulated (Fig. 2b ). Consistent with a role of IRF-1 as negative regulator of cell cycle and cell proliferation, genes related to DNA-binding ( Trp63 ) as well as several transcription factors ( Lhx1 , Tcf24 ) and the stem cell marker Lgr5 were among the highly upregulated genes in Irf1 –/– mice. The group of the most downregulated genes included interferon-stimulated genes such as Gbp2 , Ido1 , Ifit2 , Gbp11 , Ifit1bl1 or Gbp8 . Interestingly, the expression of several genes involved in antibacterial defense mechanisms (e.g. AW112010 [18] ) and IL-12 responses such as Tlr11 and Tlr12 , which induce the production of IL-12 in DCs [19] as well as the IL-12 receptor subunit IL12rb1 were also downregulated in the absence of IRF-1 (Fig. 2c ). Interestingly, bulk RNAseq analysis of either purified immune cells or epithelial cells separated from colons of the same C. rodentium infected mice identified Irf1 -dependend gene expression programs in both intestinal cell compartments. Notably, the numbers of differentially expressed genes between Irf1 –/– and Irf1 +/+ mice (log2 fold change >2; padj <0.05) was substantially higher in the immune cell compartment (Fig. 2d–f ). Fig. 2: Analysis of Irf1-dependent transcriptional changes during C. rodentium infection. a–c Expression profiling by bulk RNAseq of distal whole colonic tissue of C. rodentium infected Irf1 –/– and Irf1 +/+ mice (9 dpi). d–f Colonic tissue of C. rodentium infected mice (9 dpi) was removed and the epithelial and immune cell compartment was enriched as described in the methods section. Total RNA was isolated and used for expression profiling by bulk RNAseq analysis. e , f Genes showing log2 fold-changes in expression of >2 or –2 and false discovery rates (FDR) < 0.05 as determined by the Deseq2 algorithm were colored in red. Full size image Given that IRF-1 is well known to molecularly act downstream of IFN-γ signaling, we also subjected mice lacking IFN-γ to C. rodentium infection. However, compared to control mice, we observed no marked weight loss and no increased gut pathogen loads in these animals (Supplementary Fig. 1 B,C ). Although we observed a tendency towards an increased systemic spread, dissemination was much lower when compared to infected Irf1 –/– mice (Supplementary Fig. 1D ) indicating that molecular mechanisms beyond type 2 interferon signaling contribute to the protective function of IRF-1 during C. rodentium infection. Collectively, our data indicate that the transcription factor IRF-1 essentially contributes to effective C. rodentium eradication and prevents potentially fatal systemic spread in this model. Hematopoietic but not intestinal epithelial specific IRF-1 expression is required for effective control of C. rodentium infection Immunohistochemical stainings demonstrated that IRF-1 expression is strongly upregulated in both intestinal epithelial cells as well as lamina propria infiltrating immune cells in the context of C. rodentium infection (Fig. 1a ). To discriminate between hematopoietic and non-hematopoietic contributions of IRF-1 expression during C. rodentium infection, we therefore next generated bone marrow chimeric mice by reconstituting lethally irradiated C57BL/6 mice with bone marrow from Irf1 –/– or Irf1 +/+ mice and performed infection experiments eight weeks after reconstitution. Interestingly, C57BL/6 chimeras that received Irf1 –/– bone marrow suffered from marked wasting disease, while weight loss in the group of mice that were reconstituted with Irf1 +/+ bone marrow was negligible (Fig. 3a ). On day nine post infection, we observed systemic dissemination in all mice that had been reconstituted with Irf1 –/– bone marrow, while spread in the control group was significantly lower (Fig. 3b ) suggesting that Irf1 expression in the hematopoietic compartment is required to provide the host with the capacity to mount an efficient C. rodentium directed immune response. To further verify these results, we generated mice with conditional Irf1 -deficiency in the hematopoietic and endothelial ( Irf1 ΔTie2 ) and in the intestinal epithelial ( Irf1 ΔIEC ) compartments and compared the systemic spread of C. rodentium after infection in these mice. Our data clearly showed that Irf1 ΔTie2 mice had higher systemic pathogen loads than Irf1 fl/fl , Tie2 Cre Irf1 +/– control and Irf1 ΔIEC mice (Fig. 3 c,d ). Thus, IRF-1 expression in hematopoietic cells is required to prevent early bacterial overgrowth and systemic dissemination. Conversely, IRF1- expression in IECs seems to be less important in this setting, although expression of Irf1 in IECs was highly upregulated in C. rodentium -infected C57BL/6 mice. Fig. 3: IRF-1 expression is required in hematopoietic cells during C. rodentium infection. a , b Chimeric mice were generated by reconstitution of irradiated C57BL/6 mice with Irf1 +/+ or Irf1 –/– bone marrow. 8 weeks later, chimeras were infected with C. rodentium and analyzed 9 dpi. a Weights are shown as percentage of baseline ( Irf1 +/+ BM: n = 13, Irf1 –/– BM: n = 11). b C. rodentium dissemination to livers, spleens and mLNs. ( Irf1 +/+ BM: n = 10, Irf1 –/– BM: n = 5). c Irf1 –/– , Irf1 ΔTie2 and Irf1 ΔIEC mice were infected with C. rodentium and compared to Irf1 fl/fl mice. ( Irf1 ΔTie2 : n = 12, Irf1 ΔIEC : n = 8, Irf1 fl/fl : n = 18, Irf1 –/– : n = 5) d Tie2 Cre+ Irf1 fl/fl mice were infected and compared to Tie2 Cre+ Irf1 fl/wt control mice ( Tie2 Cre+ Irf1 fl/fl : n = 6, Tie2 Cre+ Irf1 fl/wt : n = 5). Data is expressed as mean ± SEM. Exact p values defined by two-tailed Mann–Whitney U test ( a , b , d ) or by one-way ANOVA (Kruskal Wallis test) with Dunnett’s multiple comparisons test ( c ). Source data are provided as a Source data file. Full size image IRF-1 deficiency impairs the effector functions of innate lymphoid cells during C. rodentium infection Characteristic cytokine secretion patterns of hematopoietic cells play essential roles during C. rodentium directed mucosal immunity [20] . To decipher the protective role of IRF-1 during the immune response against this pathogen in more detail, we next compared colonic cytokine expression profiles in infected Irf1 –/– and control mice at 8 dpi by specific qPCR analysis. While transcript numbers of IL-17A were comparable between control and Irf1 -deficient mice, the transcripts of IFN-γ and particularly IL-22 were reduced in the absence of IRF-1 (Fig. 4a ). Likewise, serum concentrations of IL-22 and IFN-γ, but not of IL-17A were significantly reduced in Irf1 –/– mice in comparison to controls (Fig. 4b ). Notably, we observed a similar reduction of IFN-γ and IL-22 on mRNA and protein level in C. rodentium infected Irf1 ΔTie2 mice compared to Irf1 fl/fl (Fig. 4c, d ) or Tie2 Cre Irf1 fl/wt mice (Fig. 4e ) as well as in chimeric mice reconstituted with bone marrow cells of Irf1 –/– mice (Fig. 4f ). By contrast, Irf1 ΔIEC mice exhibited similar IL-22 serum levels as Irf1 fl/fl controls. Fig. 4: Irf1 deficiency impairs IL-22 and IFN-γ secretion during C. rodentium infection. a , b Irf1 –/– and control mice were infected with C. rodentium . a Total RNA of distal colonic tissue (8 dpi) was analyzed by specific qRT-PCR. ( Il17 , Ifng : Irf1 +/– : n = 8, Irf1 –/– : n = 7; Il22 : Irf1 +/– : n = 12, Irf1 -/– : n = 9). b Serum-concentrations of IL-17A, IFN-γ and IL-22 were measured by specific ELISAs. (IL-17: Irf1 +/– : n = 10, Irf1 -/– : n = 11; IFN-γ: Irf1 +/– : n = 10, Irf1 –/– : n = 10; IL-22: Irf1 +/– : n = 12, Irf1 –/– : n = 8). c , d , e Irf1 ΔTie2 and littermate control mice were infected with C. rodentium . c Total RNA of distal colonic tissue (8 dpi) was analyzed by specific qRT-PCR. ( Il17: Irf1 fl/fl : n = 14, Irf1 ΔTie2 : n = 12;, Ifng : Irf1 fl/fl : n = 13, Irf1 ΔTie2 : n = 12; Il22 Irf1 fl/fl : n = 12, Irf1 ΔTie2 : n = 13). d Serum-concentrations of IL-17A, IFN-γ and IL-22 were measured by specific ELISAs. (IL-17: n = 14/group, IFN-γ: Irf1 fl/fl : n = 13, Irf1 ΔTie2 : n = 12, IL-22: Irf1 fl/fl : n = 12, Irf1 ΔTie2 : n = 14). e Serum-concentrations of IL-17A, IFN-γ and IL-22 were measured by specific ELISAs. (IL-17, IL-22: Irf1 fl/+ Tie2cre + : n = 5/group, Irf1 fl/fl Tie2cre + : n = 6, IFN-γ: Irf1 fl/+ Tie2cre + : n = 5, Irf1 fl/fl Tie2cre + : n = 5). f Chimeric mice were generated by reconstitution of irradiated C57BL/6 mice with Irf1 +/+ or Irf1 –/– bone marrow. 8 weeks later, chimeras were infected with C. rodentium and serum-concentrations of IL-17A, IFN-γ and IL-22 were measured by specific ELISAs (9 dpi). (IL-17, IFN-γ: Irf1 +/+ : n = 8, Irf1 –/– : n = 3; IL-22: Irf1 +/+ : n = 10, Irf1 –/– : n = 4). Data is expressed as mean ± SEM. Exact p values defined by two-tailed Mann–Whitney U test are provided in the plots. Source data are provided as a Source data file. Full size image Both T cells and innate lymphoid cells (ILCs) have been shown to be important producers of IL-22 and IFN-γ during C. rodentium infection [21] , [22] , [23] . To characterize the differences in the expression patterns of these cytokines on a cellular level, we conducted flow cytometry analysis using colonic lamina propria mononuclear cells (LPMCs) of infected Irf1 –/– and Irf1 +/– control mice. In accordance with previous reports [24] , we observed reduced frequencies of T H 1 cells (lin + Thy1 + Tbet + cells) in Irf1 –/– LPMCs. Interestingly, the frequencies of RORγt-expressing T cells (lin + Thy1 + RORγt + cells), which include T H 17 and T H 22 cells, were also reduced in these mice. However, intracellular cytokine stainings did not detect IRF-1-dependend differences in their capability to produce IL-22 and IFN-γ (Supplementary Fig. 1E, F, G ). Within the innate lineage however, the frequencies of Tbet-expressing ILCs (lin - Thy1 + Tbet + cells) (Fig. 5a ), ILC1s (lin - Thy1 + Tbet + EOMES - NK1.1 + NKp46 + ) (Fig. 5b ) and RORγt-expressing ILC3s (lin - Thy1 + RORγt + ) producing IL-22 (Fig. 5c ) were reduced in Irf1 –/– LPMCs compared to controls. In line with these findings, the abundances of IFN-γ- and IL-22-expressing ILCs were also significantly reduced in Citrobacter infected Irf1 ΔTie2 mice (Fig. 5d ). Because, the mouse intestinal lamina propria contains substantial numbers of ILC2s, we also analyzed the impact of Irf1 -deficiency on this particular ILC subset. However, we observed no statistically significant differences between both genotypes in the steady state and in the context of C. rodentium infection (Fig. 5e ). Fig. 5: Irf1 expression regulates cytokine responses of intestinal innate lymphoid cells. a–d Irf1 –/– and Irf1 +/– control or Irf1 ΔTie2 and Irf1 fl/fl control mice were infected with C. rodentium . LPMCs were isolated at 8 dpi and analyzed by flow cytometry. Graphs show relative abundances and frequencies of Tbet + ILCs (lin - Thy1.2 + Tbet + ), IFN-γ producing Tbet + ILCs (lin - Thy1.2 + Tbet + IFN-γ + ), ILC1s (lin - Thy1.2 + Tbet + EOMES - NK1.1 + Nkp46 + ) as well as relative abundances and frequencies of RORγt + ILC3s (lin - Thy1.2 + RORγt + ) and ILC3s expressing IL-22 (lin - Thy1.2 + RORγt + IL-22 + ). a n = 5/group; ( b ) n = 3/group; ( c ) Irf1 +/– : n = 8, Irf1 +/– : n = 9. d Irf1 fl/fl : n = 9, Irf1 ΔTie2 : n = 8. e Comparison of intestinal ILC2 frequencies in Irf1 –/– and Irf1 +/– control mice in the steady state or in the context of C. rodentium infection (CR); n = 3/group. Data is expressed as mean ± SEM. Exact p values defined by two-tailed Mann–Whitney U test are provided in the plots. Source data are provided as a Source data file. Full size image Next, we adoptively transferred bone marrow of control or Irf1 –/– mice (both CD45.2 + ) to irradiated recipient mice harboring the congenic marker CD45.1 to allow discrimination of donor ILCs from radioresistant ILCs (Supplementary Fig. 2A ). These experiments demonstrated that C. rodentium infected mice receiving Irf1 –/– bone marrow had significantly lower frequencies of intestinal IL-22 producing ILC3s, while Tbet + ILCs were less affected. Supplementary Fig. 2B-D ). Although ILC3s in general require the transcription factors RORγt and AHR for development, phenotypically and functionally distinct subsets exist in the intestinal lamina propria [1] , [25] . In mice, the two best characterized groups can be distinguished by their expression of the chemokine receptor CCR6 and the natural cytotoxicity receptor NKp46 [4] , [5] . Given the significant reduction of IL-22-producing ILC3s in Irf1 –/– mice, we therefore next analyzed, whether Irf1 -deficiency differentially disturbs ILC3 subsets in the gut lamina propria. Already under steady state conditions, the relative abundance of CCR6 - NKp46 + ILC3s was reduced in Irf1 –/– mice, while there were no significant changes in the frequencies of CCR6 + NKp46 - ILC3s in LPMCs of Irf1 –/– mice (Supplementary Fig. 3A ). Similarly, the numbers of CCR6 - NKp46 + ILC3s were drastically reduced in the absence of IRF-1 in the context of C. rodentium infection (Supplementary Fig. 3B ). The absolute numbers of CCR6 + NKp46 - ILC3s were also reduced in Irf1 –/– mice indicating that IRF-1 transcription controls cellularity of both ILC3 subsets during infection (Supplementary Fig. 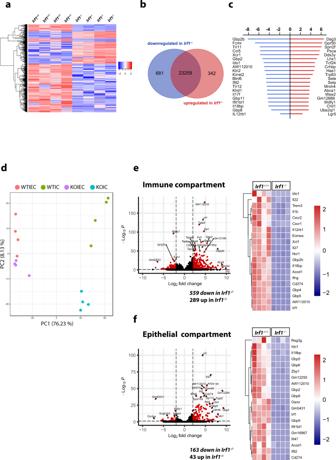Fig. 2: Analysis of Irf1-dependent transcriptional changes during C. rodentium infection. a–cExpression profiling by bulk RNAseq of distal whole colonic tissue ofC. rodentiuminfectedIrf1–/–andIrf1+/+mice (9 dpi).d–fColonic tissue ofC. rodentiuminfected mice (9 dpi) was removed and the epithelial and immune cell compartment was enriched as described in the methods section. Total RNA was isolated and used for expression profiling by bulk RNAseq analysis.e,fGenes showing log2 fold-changes in expression of >2 or –2 and false discovery rates (FDR) < 0.05 as determined by the Deseq2 algorithm were colored in red. 3B ). Importantly, further flow cytometric analysis of LPMC after C. rodentium infection showed that all studied ILC3 subtypes of Irf1 –/– mice (CCR6 + NKp46 - , CCR6 - NKp46 - , CCR6 - NKp46 + ) had a significantly diminished potential to produce IL-22 compared to control ILC3s (Supplementary Fig. 3C ). Because expression of the cytokine IL-23 is essential for C. rodentium -directed mucosal immunity and intestinal ILC responses [26] , we next subjected control and Irf1 –/– mice to systemic IL-23 treatment and compared the expression of IFN-γ, IL-22 and IL-17A in this setting. Expectedly, IL-22 and IFN-γ were hardly detectable under steady state conditions. However, IL-23 treatment resulted in a strong increase of IL-22 and IFN-γ transcripts and protein in control mice, while this upregulation was blunted in Irf1 –/– mice (Fig. 6 a,b ). Noteworthy, similar to the data in C. rodentium infected mice, the frequencies of Tbet + IFN-γ-expressing and Rorγt + IL-22-expressing ILCs were reduced in the absence of IRF-1 (Fig. 6 c,d ). To more specifically analyze the cytokine responses of these cells in vitro, we flow-sorted lamina propria ILCs of Citrobacter -infected control and Irf1 –/– mice. Consistent with our previous flow cytometric data using LPMC, much less absolute numbers of ILCs were recovered from intestines of Irf1 -deficient mice compared to controls ( Fig. 6e ). Although the expression of IL-22 and IFN-γ was very low in unstimulated ILCs, stimulation of control ILCs with a combination of IL-23 and IL-1β led to induction of IL-22 and to a lesser extend IFN-γ expression at both the RNA level (Fig. 6f , Supplementary Fig. 4A ) and protein level (Fig. 6g , Supplementary Fig. 4B ). By contrast, the induction of IL-22 and IFN-γ expression was strongly attenuated in Irf1 –/– ILCs upon stimulation of the same number of ILCs (Fig. 6f, g, h ). Conversely, the stimulation-dependent secretion of IL-17A was not altered in Irf1 +/– and Irf1 –/– ILCs indicating that cell death is not a primary driver of the observed differences in cytokine expression patterns. Fig. 6: Irf1-/- ILCs fail to produce IL-22 and IFN-γ due to a cell intrinsic defect. a–d Irf1 +/– and Irf1 –/– mice were challenged with an IL-23-expression vector for three days. a The expression of Ifng , Il22 and Il17a in gut tissue samples was quantified by qRT-PCR with total RNA ( Il17 : Irf1 +/– untreated n = 6, IL-23 n = 11; Irf1 –/– untreated n = 5, IL-23 n = 11; Ifng : Irf1 +/– untreated n = 6, IL-23 n = 11; Irf1 –/– untreated n = 6, IL-23 n = 11; Il22 : Irf1 +/– untreated n = 5, IL-23 n = 10; Irf1 –/– untreated n = 5, IL-23 n = 11) and ( b ) serum-concentrations of IFN-γ, IL-22 and IL-17a were measured by specific ELISAs (IL-17: Irf1 +/– untreated n = 7, IL-23 n = 11; Irf1 –/– untreated n = 6, IL-23 n = 10; IFN-γ: Irf1 +/– untreated n = 7, IL-23 n = 11; Irf1 –/– untreated n = 6, IL-23 n = 10; IL-22: Irf1 +/– untreated n = 6, IL-23 n = 11; Irf1 –/– untreated n = 6, IL-23 n = 10). c , d Intestinal LPMCs were isolated and analyzed by flow cytometry. Graphs show frequencies of Tbet + ILCs (lin - Thy1.2 + Tbet + cells), ILC1s (lin - Thy1.2 + Tbet + EOMES - NK1.1 + Nkp46 + ), ROR-γt + ILC3s (lin - Thy1.2 + RORγt + cells) and of ILC3s expressing IL-22 ( Irf1 +/– : n = 4, Irf1 –/– : n = 3). e–h Irf1 +/– and Irf1 –/– ILCs were sort-purified from LPMC before in vitro stimulation ( n = 3/group). e Numbers of input cells and the yield of sort-purified ILCs (CD45 + B220 - CD3 - CD5 - CD11b - CD11c - KLRG1 - CD127 + Thy1.2 + cells) are shown. f–h ILCs were stimulated with IL-1β (20 ng/ml) and IL-23 (20 ng/ml) or left unstimulated (medium). f Total RNA of ILCs was analyzed by specific qRT-PCR. g After 72 h, supernatants were collected to measure concentrations of IL-17A, IL-22 and IFN-γ by ELISA. h IL-22 production of RORγt + ILCs was studied by flow cytometry. Data is expressed as mean ± SEM. Exact p-values defined by 2way ANOVA with Tukey´s multiple comparisons test are provided in the plots. n.d.: not detectable. Source data are provided as a Source data file. Full size image Collectively, these data indicate that Irf1 -deficiency in the hematopoietic compartment is associated with a reduced capacity of intestinal lymphocytes to produce IL-22 and IFN-γ upon infection or IL-23 challenge. This phenotype is specifically linked to altered numbers and activation patterns within subsets of intestinal innate lymphoid cells in these mice. IRF-1 controls IL-23-dependent activation of intestinal ILC3s via IL-12Rβ1 In order to better define IRF-1-dependent transcriptional regulation of gut ILCs, we performed RNA-seq of FACS-sorted lamina propria ILC1/ILC3s of C. rodentium -infected Irf1 –/– and Irf1 +/– control mice. Principal component analysis showed that IRF-1-deficient ILCs clustered separately from their wild-type counterparts, demonstrating a unique role of IRF-1 in determining their transcriptome (Supplementary Fig. 5A ). We identified more than 1000 genes (691 downregulated, 592 upregulated in Irf1 –/– ) as differentially expressed (FC > 2, adjp-value <0.05) between Irf1 –/– and control ILCs (Supplementary Fig. 5B ). The list of highly downregulated genes includes several IFN-inducible genes such as AW112010 , Gbp2 , Iigp1 , Gm4951 and F830016B08RiK , but also genes previously implicated in ILC functions such as Cysltr2 and Csf2 . Consistent with our flow cytometry data, we detected a downregulation of IL22 transcripts in the absence of IRF-1. (Supplementary Fig. 5C ). Furthermore, KEGG and GO enrichment analysis of differentially expressed genes (DEGs) between control and Irf1 -/- ILCs suggested that several DEGs are associated with important immune-related pathways including ‘Cytokine-cytokine receptor interaction’ (Supplementary Fig. 5D ). The cell surface receptor IL-12Rβ1 forms with IL-12Rβ2 the receptor for the cytokine IL-12 or interacts with IL-23R to constitute a functional IL-23 receptor [27] . Interestingly, our RNA-Seq analysis of both sorted intestinal ILC3s and immune cells of C. rodentium infected mice clearly showed that the expression levels of Il12rb1 were strongly reduced in Irf1 –/– mice. Because IL-12 and IL-23 receptor signaling have been shown to be central regulators of human ILC plasticity [28] and IRF-1 transactivates the Il12rb1 gene promoter in CD4 + T cells [29] , we compared the expression of this shared receptor chain in intestinal tissue of control and Irf1 –/– mice by qPCR. These data confirmed that Il12rb1 expression was profoundly reduced in Irf1 –/– mice, while the transcripts of Il12rb2 and Il23r were comparable between both groups of mice (Fig. 7a ). Moreover, flow cytometric analysis clearly demonstrated that the presence of IRF-1 is required for IL-12rβ1 expression on intestinal ILC3s (Fig. 7b ), while the IL-23R chain was similar in control and Irf1 –/– mice (Fig. 7c ). Fig. 7: Reduced expression of IL12rb1 in Irf1-deficient intestinal ILC3s. Irf1 +/ – and Irf1 –/– mice were infected with C. rodentium and were sacrificed eight days post infection. a Quantification of Il12rb1 ( Irf1 +/– : n = 13, Irf1 –/– : n = 10), Il12rb2 ( Irf1 +/– : n = 17, Irf1 –/– : n = 12) and Il23r ( Irf1 +/– : n = 12, Irf1 –/– : n = 10) transcripts in total RNA of distal colon tissue samples by specific qRT-PCR. b , c Flow cytometric analysis of IL-12Rβ1 ( n = 5/group) and IL-23R ( Irf1 +/– : n = 4, Irf1 –/– : n = 3)-expressing ILC3s (lin - Thy1.2 + RORγt + cells). Data is expressed as mean ± SEM. Exact p– values defined by two-tailed Mann-Whitney U test are provided in the plots. Source data are provided as a Source data file. Full size image Collectively, these data indicate that IRF-1 is a critical regulator of intestinal ILC3 numbers and their functional potential by regulation of IL-12rβ1. IL-22 treatment protects Irf1 –/– mice from systemic C. rodentium dissemination In the first days after infection, ILC3s provide protection from C. rodentium -dependent disease [30] . Given the profound changes in the ILC3 compartment in Irf1 –/– mice, we next aimed to specifically address the contribution of ILC3 intrinsic Irf1 expression to disease manifestation. We therefore generated mixed bone marrow chimeric mice lacking Irf1 in ILC3s by adoptive transfer of bone marrow cells of ILC3-deficient Rorgt –/– mice and Irf1 −/− mice mixed at a ratio of 80:20 [31] into irradiated, lymphopenic Rag2 –/– IL2rγ –/– mice (Fig. 8a ). Control chimeras received 20% WT bone marrow in place. In these chimeras, all ILC3s were either WT or Irf1 -deficient, while the majority of other hematopoietic and non- hematopoietic cells were Irf1 -sufficient. At 8 dpi after C. rodentium treatment, IL-22 + ILC3s were reduced in mice receiving Irf1 –/– bone marrow (Fig. 8b ) and accordingly, serum IL-22 concentrations were reduced (Fig. 8c ). Moreover, these mice displayed higher systemic spread than controls receiving Irf1 -proficient ILC3s (Fig. 8d ) supporting the notion that Irf1 -expression in ILC3s directly supports C. rodentium directed defense mechanisms. IL-22 production by ILCs has emerged as a central protective mechanism in the early phase of the C. rodentium infection model. Within ILCs, this function has been largely assigned to Lti-like CCR6 + ILC3s and their capacity to produce large amounts of IL-22 upon stimulation, while NKp46 + ILC3s producing IFN-γ were redundant even in the absence of T cells [32] , [33] . We therefore inferred that rather their strong ILC3-intrinsic defects to produce IL-22 than the lack of NKp46 + ILCs supports the observed fatal systemic spread in Irf1 –/– mice. To directly test this hypothesis, we increased the systemic abundance of IL-22 [34] in Irf1 –/– and control mice and compared the disease outcome with untreated mice. C. rodentium detection by immunohistochemical staining clearly demonstrated colonization of deep colonic crypt spaces in untreated Irf1 –/– mice compared to Irf1 -proficient mice at day 7 post infection. Conversely, the pathogen was restricted to the top of the colonic crypts in Irf1 -/- and control mice subjected to IL-22 treatment (Fig. 8e ). Moreover, IL-22 treatment almost completely prevented systemic C. rodentium spread even in the absence of IRF-1 as evidenced by analysis of tissue homogenates on selective agar plates (Fig. 8f ) highlighting the essential impact of this cytokine for pathogen containment to the gut lumen. Fig. 8: IL-22 treatment protects Irf1 –/– mice from systemic C. rodentium dissemination. a Mixed bone marrow (BM) chimeras with 80% RORγt –/– (ILC3 deficient) and 20% control or Irf1 –/– bone marrow were generated. After 8 weeks, mice were infected with C. rodentium and analyzed at 8 dpi. b Flow cytometric analysis of ILC3s (lin - Thy1.2 + RORγt + ) and ILC3s expressing IL-22 ( n = 3/group). c Serum IL-22 concentrations were measured by specific ELISA ( n = 5/group). d Dissemination of C. rodentium was analyzed by determination of CFU/g tissue from livers, spleens and mLNs ( n = 5/group). e , f Control and Irf1 –/– mice were injected with an Il22 expression vector. After three days, mice were infected with C. rodentium . e C. rodentium colonization of the colonic epithelial surface was visualized by staining of colonic cross sections. Scale bars represent 50 µm. f Dissemination of C. rodentium was analyzed by determination of CFU/g tissue from livers ( Irf1 +/– : untreated n = 7, IL-22 n = 5; Irf1 –/– : n = 3/group), spleens ( Irf1 +/– : untreated n = 6, IL-22 n = 5; Irf1 –/– : n = 3/group) and CFU/ml blood ( Irf1 +/– : untreated n = 6, IL-22 n = 5; Irf1 –/– : n = 3/group). Data is expressed as mean ± SEM. Exact p values defined by two-tailed Mann–Whitney U test ( b – d ) or 2way ANOVA with Tukey’s multiple comparisons test ( f ) are provided in the plots. Source data are provided as a Source data file. Full size image In conclusion, this study provides further insights into the function of the transcription factor IRF-1 during enteric infections and potentially other gut diseases such as IBD. Even though IRF-1 is known to be an important driver of type 1 immunity against intracellular pathogens, we were able to show here that this transcription factor also plays indispensable tasks during type 3 immune responses following A/E enteropathogenic infection of the large intestine. In this context, we identified IRF-1 by analysis of conventional and novel conditional gene-deficient mice as central regulator of ILC1 and ILC3 cellularity and their capacity to produce prototypic cytokines. Thereby, IRF-1 expression was of particular importance for activation-dependent production of IL-22 by both CCR6 + NKp46 - and CCR6 - NKp46 + ILC3 subsets, which was related to prevention of C. rodentium dissemination. Mechanistically, our data indicate that IRF-1 signaling stimulates the expression of the shared IL-12Rβ1 chain in ILCs thereby providing ILC3s the capacity to respond to the cytokines IL-12 and IL-23, which are abundantly produced by myeloid cells in the course of enteric infections [35] , [36] . Previously, IRF-1 has been implicated in various effector functions of T cells including CD8 + T cells, Tr1 cells and Th1 cells [11] . Kano et al. found that differentiation of naive CD4 + T cells into IFN-γ producing Th1 cells was directly linked to IRF-1 binding to the IL12Rb1 gene promoter, while Th17 cell differentiation was not affected in Irf1 –/– mice [29] . A potential mechanism to explain this differential requirement of IRF-1-dependent regulation of IL12rb1 is that less IL-12Rβ1 is sufficient for IL-23-signaling, while higher levels are required for IL-12-induced Th1 differentiation. In line with this study, we found decreased frequencies of intestinal Th1 cells in infected Irf1 -/- mice, while the production of IL-22 and IL-17 by T cells was not profoundly affected. Conversely, our in vitro and in vivo data clearly indicate that the IL-23-dependent production of IL-22 strongly depends on the presence of IRF-1. IL-22 is a central mediator of protective immunity towards C. rodentium infection. While IL-22 release from both innate and adaptive cells is required for effective eradication of this pathogen [22] , ILC3s represent the main source of IL-22 in the early phase of infection [7] . The early severe phenotype of Irf1 –/– mice in this model together with the fact that ectopic IL-22 expression alone was sufficient to provide complete protection clearly suggest that IRF-1-dependent expression of IL-22 is critical for mucosal clearance of extracellular bacterial pathogens and reestablishment of homeostasis. However, although our study also identified IRF-1 as important fine tuner of the accumulation of intestinal NCR + ILC subsets producing IFN-γ, these data support previous studies showing that NCR + ILC3s are redundant in the context of C. rodentium infection [32] , [33] . Given their reported host protective functions e.g. during infections with Salmonella enterica [4] , Toxoplasma gondii [37] or viral infections [38] , it therefore remains interesting to study the contribution of IRF-1 dependent IFN-γ producing ILCs in these models. It also still needs to be investigated, whether IRF-1 signaling supports pathogenic functions of IL-22 and IFN-γ producing ILC3s that have been reported in e.g. anti-CD40-induced innate colitis [39] , [40] , [41] . Future fate-mapping approaches and scRNA and/or scATAC-seq studies using wildtype and Irf1 -deficient mice will help to provide a more comprehensive understanding of the function of IRF1 signaling for the transcriptional regulation of intestinal ILC plasticity and the identification of transcriptional targets in individual ILC populations including ILC1, exILC3 and different ILC3 subsets. Noteworthy, the human IRF-1 gene is located in the IBD5 susceptibility locus on chromosome 5, which is a risk haplotype associated with Crohn’s disease [42] . Thus, IRF-1 signaling may also be implicated in progression and aggravation of inflammatory bowel diseases by supporting the accumulation of dysregulated NCR + ILCs, which has been reported in the inflamed gut mucosa in CD [43] , [44] . Animals and housing conditions Irf1 –/– mice [45] were kindly provided by A. Kröger (University of Magdeburg). Irf1 –/– mice were bred with Irf1 +/– as littermate controls or were co-housed with Irf1 +/+ mice for at least four weeks to ensure adaptation of the intestinal microbiome. No evident differences in α and β-diversity of the intestinal microbiota could be detected by 16S-based metagenomic sequencing (Supplementary Fig. 6A, B ). Ifng -/- mice were originally purchased from the Jackson Laboratory and were bred in-house. Irf1 fl/fl mice were generated in-house through crossing a mouse strain purchased from the European Mouse Mutant Archive (EMMA) of the European Conditional Mouse Mutagenesis Program (EUCOMM) with a general FLP deleter strain. Irf1 fl/fl mice were crossed to Tie2-cre mice or Villin-cre mice (Jackson Laboratory) to generate Irf1 ΔTie2 and Irf1 Δ IEC mice respectively. All mice were bred on a C57BL/6 background and kept in individually ventilated cages. Mice of different experimental groups were age- and sex-matched. Sterile drinking water and food were provided ad libitum . Animal husbandry and experimental procedures were approved by the Government of Unterfranken (55.2.2-2532-2-712). C. rodentium infection model and quantification of the bacterial burden To analyze the relevance of IRF-1 during infectious colitis, mice were infected with an erythromycin resistant and luminescent strain of Citrobacter rodentium ( C. rodentium; strain ICC169) kindly provided by Christian Riedel [46] . Prior to infection, mice were fasted for 8 hours. C. rodentium was cultivated in sterile, erythromycin-supplemented (500 µg/ml) LB-medium at 37 °C with shaking and used for infection during the phase of exponential growth. For infection, bacteria were resuspended in sterile PBS and mice were inoculated with ~4 × 10 9 CFU of C. rodentium in 200 µl PBS by oral gavage using a feeding needle. For analysis of bacterial burdens, C. rodentium luminescence was measured by in vivo-imaging using an IVIS Spectrum CT system (PerkinElmer, Waltham, Massachusetts). Therefore, the abdomen of the infected mice was depilated and they were anesthetized with 1,5-2% isoflurane. 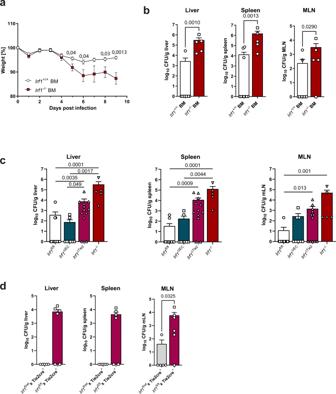Fig. 3: IRF-1 expression is required in hematopoietic cells duringC. rodentiuminfection. a,bChimeric mice were generated by reconstitution of irradiated C57BL/6 mice withIrf1+/+orIrf1–/–bone marrow. 8 weeks later, chimeras were infected withC. rodentiumand analyzed 9 dpi.aWeights are shown as percentage of baseline (Irf1+/+BM:n= 13,Irf1–/–BM:n= 11).bC. rodentiumdissemination to livers, spleens and mLNs. (Irf1+/+BM:n= 10,Irf1–/–BM:n= 5).cIrf1–/–,Irf1ΔTie2andIrf1ΔIECmice were infected withC. rodentiumand compared toIrf1fl/flmice. (Irf1ΔTie2:n= 12,Irf1ΔIEC:n= 8,Irf1fl/fl: n = 18,Irf1–/–:n= 5)dTie2Cre+Irf1fl/flmice were infected and compared toTie2Cre+Irf1fl/wtcontrol mice (Tie2Cre+Irf1fl/fl:n= 6,Tie2Cre+Irf1fl/wt:n= 5). Data is expressed as mean ± SEM. Exactpvalues defined by two-tailed Mann–Whitney U test (a,b,d) or by one-way ANOVA (Kruskal Wallis test) with Dunnett’s multiple comparisons test (c). Source data are provided as a Source data file. Quantification of luminescence was performed using the IVIS-associated software Living Image 4.0 . For determination of C. rodentium in feces, fresh stool samples were collected and weighed. To quantify C. rodentium CFUs in liver, spleen or mLN, fresh tissue samples were weighed, covered with LB medium (1 ml LB medium per 0.1 g tissue) and homogenized in a mixer mill (MM 400, Retsch, Germany) at a frequency of 25 Hz for 2 min. Serial dilutions of dissolved stool pellets, blood or tissue homogenates were plated on erythromycin-supplemented LB-Agar plates. After an incubation time of 20 h at 37 °C, C. rodentium colonies were counted. Bone marrow chimeric mice For the generation of bone marrow chimeric mice, lethally irradiated (10 Gray) C57BL/6 mice or congenic B6.SJL mice were reconstituted with 1 × 10 7 femoral bone marrow cells of either Irf1 +/+ mice or Irf1 -/- mice via i.v. injection. In some experiments, Rag2 –/– γc –/– were irradiated with a dose of 5 Gray and i.v. transferred with mixed donor bone marrow containing 80% Rorgt –/– and 20% wildtype or Irf1 –/– bone marrow cells. Reconstituted mice were treated with antibiotics (Borgal, Virbac, France) for 2–3 weeks to prevent infections in the recovery phase. Eight weeks after hematopoietic reconstitution, bone marrow chimeric mice were analyzed in the steady state or infected with C. rodentium . Isolation of lymphocytes from the lamina propria and from mesenteric lymph nodes Single cell suspensions from mesenteric lymph nodes were prepared through digestion with Collagenase B (0.25 mg/ml; Roche) and DNase I (0.05 mg/ml Roche) using a gentleMACS Octo Dissociator (program: 37c_m_SDK_1; Miltenyi Biotec) according to the manufacturer’s recommendations. For the isolation of lamina propria mononuclear cells (LPMCs) intestinal tissue was removed and cleaned from residual fat. Luminal contents were flushed out and the intestinal tissue was cut longitudinally and then laterally into pieces of 5 mm length. LPMCs were isolated with the lamina propria dissociation kit mouse from Miltenyi Biotec according to the manufacturer’s instructions under use of a gentleMACS Octo Dissociator (Miltenyi Biotec) running the program m_intestine_01. After the isolation process, the cell suspension was proceeded to Percoll gradient centrifugation (40%/80%) for purification. Epithelial cells for bulk RNAseq analysis were isolated by incubating longitudinally opened and cleaned intestinal tissue in PBS with 1 mM DTT for 10 min and subsequently in 20 ml of prewarmed HBSS with 1.5 mM EDTA for 15 min. Next, the tissue was vortexed for 1–2 min at maximum speed and intraepithelial lymphocytes were removed using Percoll gradient centrifugation (40%/80%). The pellet containing intestinal epithelial cells was centrifuged for 10 min at 400 g and the pellet was immediately subjected to RNA extraction. Flow cytometry Prior to staining with antibodies against specific intra- or extracellular markers, freshly isolated LPMCs were incubated with anti-CD16/CD32 antibodies (anti-Fc-receptor; clone 93; eBioscience) for 10 min at 4 °C to block unspecific binding. To distinguish between cells of the innate or the adaptive compartment, LPMCs were incubated with a cocktail of biotinylated lineage antibodies including anti-B220 (RA3-6B2; eBioscience, 1:50), anti-CD3 (REA641, 1:50), anti-CD5 (1:50), anti-GR1 (RB6-8C5; eBioscience, 1:50), anti-SiglecF (REA798, 1:50) and anti-Ter119 (Ter-119, 1:50) for 10 min at 4 °C. After washing, streptavidin conjugated Brilliant Violet 421 (BioLegend, 1:666) or VioBright FITC (Miltenyi Biotec, 1:100) was applied for 30 min at 4 °C in a secondary staining combined with a selection of the following antibodies used for surface staining: anti-Thy1.2 (CD90.2 in PerCP-Vio700, 1:20), anti-CCR6 (CD196 in PE, 1:20), anti-NKp46 (REA815 in FITC, 1:50), anti-Eomes (REA116 in PE, Miltenyi, 1:10), anti-NK1.1 (PK136 in BV 421, 1:20) anti-IL23R Ab (FAB16861R in AF 647, R&D Systems, 1:66) and anti-IL-12Rβ1 (CD212 in PE; BD Pharmingen, 1:20). Subsequently, cells were fixed and permeabilized using the FoxP3 Transcription Factor Staining Buffer Set (Invitrogen) according to the manufacturer’s instructions followed by intracellular transcription factor staining with fluorochrome-coupled anti-RORγt (Q31-378 in AlexaFluor 647 or BV421; BD Pharmingen, 1:80), anti Gata3 (REA174, Miltenyi Biotec, 1:10) and anti-Tbet (eBio4B10 in PE; eBioscience, 1:40) antibodies (30 min at 4 °C). For intracellular cytokine measurements, anti-IL-22 (Poly5164 in PE; BioLegend, 1:20), anti-IL-17A (TC11-18H10.1 in PE/Cyanine7; BioLegend, 1:20) and anti-IFN-γ (XMG1.2 APC; eBioscience, 1:158) antibodies were applied in combination with the transcription factor staining. In this case, cells were stimulated with Cell Stimulation Cocktail plus protein transport inhibitors (eBioscience) according to manufacturer’s instructions for 4 h prior to antibody staining. Antibodies for flow cytometry were purchased from Miltenyi Biotech, unless specified otherwise. Samples were measured on an LSRFortessa cell analyzer (BD Biosciences, FacsDiva Software version 6.1.3) and evaluated with FlowJo 10 (FlowJo LLC). The gating strategy for characterization of the various immune cell populations is outlined in Supplementary Fig. 7 . ILC sort To purify intestinal ILCs for analysis in cell culture or for RNASeq analysis, we performed fluorescence activated cell sorting using a MoFlo Astrios EQ device (Beckman Coulter) within the Core Unit Cell Sorting Erlangen. ILCs were purified using the following surface marker panel: CD45 + (REA737 in VioBlue, 1:50), B220 - (REA755 in FITC, 1;50), CD3 - (REA641 in FITC, 1:50), CD5 - (in FITC, 1:50), CD11b - (REA592 in APC-Vio770, 1:50), CD11c - (REA754 in APC-Vio770, 1:50), KLRG1 - (2F1 in APC; eBioscience, 1:158), CD127 + (IL-7Rα; A7R34 in PE; BioLegend, 1:20), Thy1.2 + (in PerCP-Vio700, 1:20). Unless specified otherwise, all antibodies used for cell sorting were purchased from Miltenyi Biotec. In vitro ILC stimulation To assay the cytokine responses of ILC3s ex vivo, ILCs were sort purified. Therefore, freshly isolated single cell suspensions from ileum, colon and mLNs of two mice of either Irf1 +/– or Irf1 –/– genotype were pooled and stained prior to cell sorting. For in vitro stimulation, 2 × 10 4 sorted CD45 + B220 - CD3 - CD5 - CD11b - CD11c - KLRG1 - CD127 + Thy1.2 + cells were plated in 200 µl DMEM GlutaMAX medium (Gibco) supplemented with 10% FBS (Gibco), 1× MEM nonessential amino acids (Gibco), 1 mM sodium pyruvate (Gibco), 20 mM Hepes (Carl Roth), 50 µM 2-mercaptoethanol (Sigma-Aldrich) and 1 % penicillin-streptomycin (Sigma-Aldrich) in the presence of 20 ng/ml recombinant mouse IL-1β (ImmunoTools) and 20 ng/ml recombinant mouse IL-23 (Miltenyi Biotec). After 24 h or 72 h, culture supernatants were harvested for determination of cytokine concentrations by ELISA and residual ILCs were lysed for isolation of RNA. Gene expression analysis Tissue pieces from distal colon or ileum were snap-frozen in liquid nitrogen and stored at −80 °C for RNA isolation. RNA was isolated from tissue using the NucleoSpin RNA Plus kit (#740984, Macherey-Nagel) according to the manufacturer’s recommendations. To analyze gene expression of sort purified ILC3s, we used the peqGOLD Micro Spin Total RNA Kit (#13-6831, VWR) following the manufacturer’s instructions. cDNA was synthesized with the Script RT-PCR kit (#PCR-511L, Jena Bioscience, Germany). Gene expression was analyzed via quantitative real-time PCR (qRT-PCR) using pre-designed QuantiTect Primer assays (Qiagen) in a CFX Connect System (Bio-Rad). 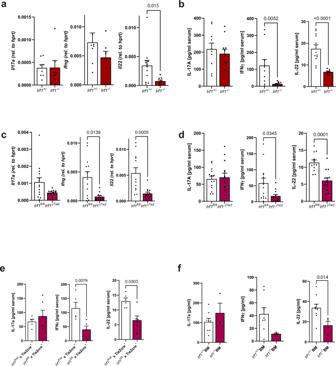Fig. 4: Irf1 deficiency impairs IL-22 and IFN-γ secretion during C. rodentium infection. a,bIrf1–/–and control mice were infected withC. rodentium.aTotal RNA of distal colonic tissue (8 dpi) was analyzed by specific qRT-PCR. (Il17,Ifng:Irf1+/–:n= 8,Irf1–/–:n= 7;Il22:Irf1+/–:n= 12,Irf1-/–:n= 9).bSerum-concentrations of IL-17A, IFN-γ and IL-22 were measured by specific ELISAs. (IL-17:Irf1+/–:n= 10,Irf1-/–:n= 11; IFN-γ:Irf1+/–:n= 10,Irf1–/–:n= 10; IL-22:Irf1+/–:n= 12,Irf1–/–:n= 8).c,d,eIrf1ΔTie2and littermate control mice were infected withC. rodentium.cTotal RNA of distal colonic tissue (8 dpi) was analyzed by specific qRT-PCR. (Il17: Irf1fl/fl:n= 14,Irf1ΔTie2:n= 12;,Ifng:Irf1fl/fl:n= 13,Irf1ΔTie2:n= 12;Il22 Irf1fl/fl:n= 12,Irf1ΔTie2:n= 13).dSerum-concentrations of IL-17A, IFN-γ and IL-22 were measured by specific ELISAs. (IL-17:n= 14/group, IFN-γ:Irf1fl/fl:n= 13,Irf1ΔTie2:n= 12, IL-22:Irf1fl/fl:n= 12,Irf1ΔTie2:n= 14).eSerum-concentrations of IL-17A, IFN-γ and IL-22 were measured by specific ELISAs. (IL-17, IL-22:Irf1fl/+Tie2cre+:n= 5/group,Irf1fl/flTie2cre+:n= 6, IFN-γ:Irf1fl/+Tie2cre+:n= 5,Irf1fl/flTie2cre+:n= 5).fChimeric mice were generated by reconstitution of irradiated C57BL/6 mice withIrf1+/+orIrf1–/–bone marrow. 8 weeks later, chimeras were infected withC. rodentiumand serum-concentrations of IL-17A, IFN-γ and IL-22 were measured by specific ELISAs (9 dpi). (IL-17, IFN-γ:Irf1+/+:n= 8,Irf1–/–:n= 3; IL-22:Irf1+/+:n= 10,Irf1–/–:n= 4). Data is expressed as mean ± SEM. Exactpvalues defined by two-tailed Mann–Whitney U test are provided in the plots. Source data are provided as a Source data file. ΔCT values were calculated to illustrate the expression of the indicated genes relative to the housekeeping gene hypoxanthine phosphoribosyltransferase 1 ( hprt ). Bulk RNAseq To analyze total transcriptome profiles of whole colon tissue (Fig. 2a–c ) after C. rodentium infection, we isolated total RNA from the distal colon of Irf1 +/+ and Irf1 -/- mice 9 d after infection. For applying the NucleoSpin RNA Plus kit (Macherey-Nagel). A total amount of 2 μg RNA per sample was used for the generation of sequencing libraries using the NEBNext Ultra RNA Library Prep Kit for Illumina (NEB) following manufacturer’s instructions. Library preparations were sequenced on an Illumina platform and paired-end reads were generated. Paired-end clean reads were mapped to the reference genome (mm10) using HISAT2 (v.2.0.5) software with default parameters [47] . FeatureCounts (v.1.6.4) was used to count the read numbers mapped to each gene [48] . Differential expression analysis between two conditions with 4 biological replicates per condition was performed using DESeq2 (v.1.22.2) [49] . The resulting p values were adjusted using the Benjamini and Hochberg’s approach for controlling the False Discovery Rate (FDR). 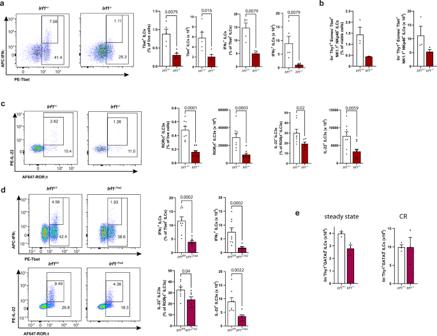Fig. 5: Irf1 expression regulates cytokine responses of intestinal innate lymphoid cells. a–dIrf1–/–andIrf1+/–control orIrf1ΔTie2andIrf1fl/flcontrol mice were infected withC. rodentium. LPMCs were isolated at 8 dpi and analyzed by flow cytometry. Graphs show relative abundances and frequencies of Tbet+ILCs (lin-Thy1.2+Tbet+), IFN-γ producing Tbet+ILCs (lin-Thy1.2+Tbet+IFN-γ+), ILC1s (lin-Thy1.2+Tbet+EOMES-NK1.1+Nkp46+) as well as relative abundances and frequencies of RORγt+ILC3s (lin-Thy1.2+RORγt+) and ILC3s expressing IL-22 (lin-Thy1.2+RORγt+IL-22+).an= 5/group; (b)n= 3/group; (c)Irf1+/–:n= 8,Irf1+/–:n= 9.dIrf1fl/fl:n= 9,Irf1ΔTie2:n= 8.eComparison of intestinal ILC2 frequencies inIrf1–/–andIrf1+/–control mice in the steady state or in the context ofC. rodentiuminfection (CR);n= 3/group. Data is expressed as mean ± SEM. Exactpvalues defined by two-tailed Mann–Whitney U test are provided in the plots. Source data are provided as a Source data file. Genes with an adjusted p value < 0.05 found by DESeq2 were assigned as differentially expressed. Cytokine measurements by Enzyme-linked immunosorbent assay (ELISA) To quantify the concentrations of IL-22, IFN-γ and IL-17A in sera and cell supernatants, Ready-SET-Go ELISA Sets from eBioscience were used according to the manufacturer’s instructions. 16 S Next generation sequencing of fecal microbiota Fecal samples were collected and immediately stored at −80 °C. Genomic bacterial DNA was isolated with the PSP Spin Stool DNA Kit (Stratec molecular, Germany) according to manufacturer’s recommendations. 10 ng of DNA was used to amplify the V3-V4 region of bacterial 16sRNA genes using the NEBNext Q5 Hot Start HiFi PCR Master Mix (NEB). Amplified PCR products were isolated with AMPure XP Beads (Beckmann Coulter Genomics), purified, pooled and subjected to 2 × 300 bp paired-end sequencing on an Illumina MiSeq platform [50] . Immunohistochemistry For immunohistochemical (IHC) stainings, distal colonic tissues from mice infected with C. rodentium were fixed in buffered formalin (Roti-Histofix; Carl Roth) at 4 °C for 24 h, dehydrated, and embedded in liquid paraffin. 3-µm sections were cut using a microtome (Leica) and processed for IHC applying the Tyramide Signal Amplification (TSA) Cy3 system (Perkin Elmer) according to the manufacturer’s protocol. To analyze the expression level of IRF-1, a primary antibody from Cell Signaling (D5E4) was used (1:50 dilution). To visualize the colonization of the mucosal surface with C. rodentium , a primary antibody from Abcam (ab37056, 1:1000) was applied. Both primary antibodies were used in combination with a goat-anti-rabbit biotinylated secondary antibody (Jackson Immuno Research). Epithelial cells were stained with Alexa Fluor 488 anti-mouse CD326 (Ep-CAM; G8.8; BioLegend, 1:100). Nuclei were counterstained with DAPI (Invitrogen). Pictures were acquired on a Leica TCS SP5 II confocal microscope using Leica LAS AF version 2.7.3.9723 software. Multiphoton microscopy Infected animals were sacrificed and fresh tissue samples from distal colons were kept in ice-cold PBS, and multiphoton microscopy (MPM) was performed on the same day. In total, 42 3D image stacks (nKO = 18, nhet = 24) were recorded and analysed from six animals ( n = 3/group). 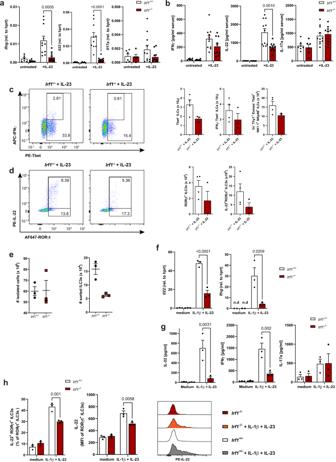Fig. 6: Irf1-/- ILCs fail to produce IL-22 and IFN-γ due to a cell intrinsic defect. a–dIrf1+/–andIrf1–/–mice were challenged with an IL-23-expression vector for three days.aThe expression ofIfng,Il22andIl17ain gut tissue samples was quantified by qRT-PCR with total RNA (Il17:Irf1+/–untreatedn= 6, IL-23n= 11;Irf1–/–untreatedn= 5, IL-23n= 11;Ifng:Irf1+/–untreatedn= 6, IL-23n= 11;Irf1–/–untreatedn= 6, IL-23n= 11;Il22:Irf1+/–untreatedn= 5, IL-23n= 10;Irf1–/–untreatedn= 5, IL-23n= 11) and (b) serum-concentrations of IFN-γ, IL-22 and IL-17a were measured by specific ELISAs (IL-17:Irf1+/–untreatedn= 7, IL-23n= 11;Irf1–/–untreatedn= 6, IL-23n= 10; IFN-γ:Irf1+/–untreatedn= 7, IL-23n= 11;Irf1–/–untreatedn= 6, IL-23n= 10; IL-22:Irf1+/–untreatedn= 6, IL-23n= 11;Irf1–/–untreatedn= 6, IL-23n= 10).c,dIntestinal LPMCs were isolated and analyzed by flow cytometry. Graphs show frequencies of Tbet+ILCs (lin-Thy1.2+Tbet+cells), ILC1s (lin-Thy1.2+Tbet+EOMES-NK1.1+Nkp46+), ROR-γt+ILC3s (lin-Thy1.2+RORγt+cells) and of ILC3s expressing IL-22 (Irf1+/–:n= 4,Irf1–/–:n= 3).e–hIrf1+/–andIrf1–/–ILCs were sort-purified from LPMC before in vitro stimulation (n= 3/group).eNumbers of input cells and the yield of sort-purified ILCs (CD45+B220-CD3-CD5-CD11b-CD11c-KLRG1-CD127+Thy1.2+cells) are shown.f–hILCs were stimulated with IL-1β (20 ng/ml) and IL-23 (20 ng/ml) or left unstimulated (medium).fTotal RNA of ILCs was analyzed by specific qRT-PCR.gAfter 72 h, supernatants were collected to measure concentrations of IL-17A, IL-22 and IFN-γ by ELISA.hIL-22 production of RORγt+ILCs was studied by flow cytometry. Data is expressed as mean ± SEM. Exact p-values defined by 2way ANOVA with Tukey´s multiple comparisons test are provided in the plots. n.d.: not detectable. Source data are provided as a Source data file. An upright Multiphoton microscope (TriMScope II, LaVision BioTec, Bielefeld, Germany) was used in combination with a water immersion objective (HC Fluortar L 16x/0.6 W VISIR, Leica microsystems, Wetzlar, Germany) and a femtosecond-pulsed Ti-Sapphire laser (Chameleon Vision II, Coherent, Santa Clara, CA, USA), at a wavelength of 810 nm. Exponential z adaptation of the laser power was used to compensate for attenuation at greater tissue depths. As previously described, the optical filters were chosen to target second harmonic generation (SGH) from collagen-I (ET405/20, Chroma, Vermont, USA), and natural autofluorescence from NADH in mucosal epithelial cells (450/70 BrightLine HC, Semrock Inc., Rochester, NY, USA) [17] . In addition to that, a third channel was used to target fluorescence from mRuby-expressed by the reporter bacteria. MPM stacks were recorded at an axial spacing of 2 µm. The lateral image size was 682 × 682 µm², separated into 512 × 512 or 1024 × 1024 pixels. The image contrast was adjusted manually using Fiji/ImageJ 1.5 upon visual inspection. No further image processing has been used. The number of bacterial clusters was counted manually in each image and divided by the area of the field of view in order to obtain the cluster density. The average cluster density per sample was calculated from all six images of the respective sample. Statistics Experimental results were plotted and analyzed for statistical significance with GraphPad Prism 8.3 (GraphPad Software Inc.), Excel 2016 and R 4.2.0. Data are shown as mean ± SEM. 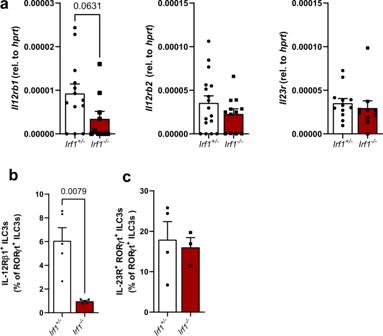Fig. 7: Reduced expression of IL12rb1 in Irf1-deficient intestinal ILC3s. Irf1+/–andIrf1–/–mice were infected withC. rodentiumand were sacrificed eight days post infection.aQuantification ofIl12rb1(Irf1+/–:n= 13,Irf1–/–:n= 10),Il12rb2(Irf1+/–:n= 17,Irf1–/–:n= 12) andIl23r(Irf1+/–:n= 12,Irf1–/–:n= 10) transcripts in total RNA of distal colon tissue samples by specific qRT-PCR.b,cFlow cytometric analysis of IL-12Rβ1 (n= 5/group) and IL-23R (Irf1+/–:n= 4,Irf1–/–:n= 3)-expressing ILC3s (lin-Thy1.2+RORγt+cells). Data is expressed as mean ± SEM. Exactp–values defined by two-tailed Mann-Whitney U test are provided in the plots. Source data are provided as a Source data file. 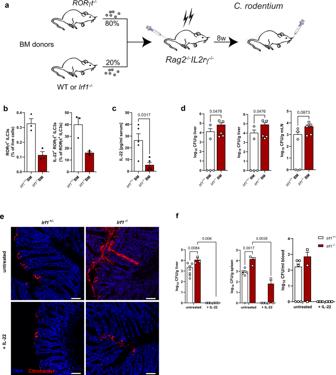Fig. 8: IL-22 treatment protects Irf1–/–mice from systemic C. rodentium dissemination. aMixed bone marrow (BM) chimeras with 80% RORγt–/–(ILC3 deficient) and 20% control orIrf1–/–bone marrow were generated. After 8 weeks, mice were infected withC. rodentiumand analyzed at 8 dpi.bFlow cytometric analysis of ILC3s (lin-Thy1.2+RORγt+) and ILC3s expressing IL-22 (n= 3/group).cSerum IL-22 concentrations were measured by specific ELISA (n= 5/group).dDissemination ofC. rodentiumwas analyzed by determination of CFU/g tissue from livers, spleens and mLNs (n= 5/group).e,fControl andIrf1–/–mice were injected with anIl22expression vector. After three days, mice were infected withC. rodentium.eC. rodentiumcolonization of the colonic epithelial surface was visualized by staining of colonic cross sections. Scale bars represent 50 µm.fDissemination ofC. rodentiumwas analyzed by determination of CFU/g tissue from livers (Irf1+/–: untreatedn= 7, IL-22n= 5;Irf1–/–:n= 3/group), spleens (Irf1+/–: untreatedn= 6, IL-22n= 5;Irf1–/–:n= 3/group) and CFU/ml blood (Irf1+/–: untreatedn= 6, IL-22n= 5;Irf1–/–:n= 3/group). Data is expressed as mean ± SEM. Exactpvalues defined by two-tailed Mann–Whitney U test (b–d) or 2way ANOVA with Tukey’s multiple comparisons test (f) are provided in the plots. Source data are provided as a Source data file. For comparison of two independent experimental groups, a two-tailed Mann–Whitney U test was used. If more than two groups were compared, one-way ANOVA (Kruskal Wallis Test) with Dunnett´s multiple comparisons test or 2way ANOVA with Tukey´s multiple comparisons test was performed. Differences of p ≤ 0.05 were considered as statistically significant indicated by asterisks (* p ≤ 0.05; ** p ≤ 0.01; *** p ≤ 0.001; **** p ≤ 0.0001). Reporting summary Further information on research design is available in the Nature Research Reporting Summary linked to this article.